A selective and efficient electrocatalyst for carbon dioxide reduction Converting carbon dioxide to useful chemicals in a selective and efficient manner remains a major challenge in renewable and sustainable energy research. Silver is an interesting electrocatalyst owing to its capability of converting carbon dioxide to carbon monoxide selectively at room temperature; however, the traditional polycrystalline silver electrocatalyst requires a large overpotential. Here we report a nanoporous silver electrocatalyst that is able to electrochemically reduce carbon dioxide to carbon monoxide with approximately 92% selectivity at a rate (that is, current) over 3,000 times higher than its polycrystalline counterpart under moderate overpotentials of <0.50 V. The high activity is a result of a large electrochemical surface area (approximately 150 times larger) and intrinsically high activity (approximately 20 times higher) compared with polycrystalline silver. The intrinsically higher activity may be due to the greater stabilization of CO 2 − intermediates on the highly curved surface, resulting in smaller overpotentials needed to overcome the thermodynamic barrier. Reduction in greenhouse CO 2 emissions from fossil fuel utilization is critical for human society [1] , [2] , [3] . Ideally, one would like to convert CO 2 produced in power plants, refineries and petrochemical plants to fuels or other chemicals through renewable energy utilization [4] , [5] , [6] . This desired solution imposes major technological challenges because CO 2 is a fully oxidized and thermodynamically stable molecule [7] , [8] . A suitable catalyst for CO 2 reduction is essential to achieve a cost-effective process with high efficiency and selectivity [9] . In the past two decades, electrocatalytic CO 2 reduction has attracted much attention because the required electricity may be obtained at a low cost from renewable energy sources, such as wind, solar, and wave [10] , [11] , [12] , [13] , [14] . Researchers have identified several potential catalysts that are able to reduce CO 2 electrochemically in aqueous electrolytes [15] , [16] , [17] , [18] , [19] , [20] . For example, Hori et al. [7] have shown that, at a potential of approximately −0.7 V versus the reversible hydrogen electrode (RHE), a polycrystalline gold electrocatalyst can deliver a current at 5.0 mA cm −2 with an efficiency of 87% towards carbon monoxide (CO) production, whereas polycrystalline copper exhibits a poor selectivity and requires a potential closer to −1.0 V (versus RHE) to achieve the same current density (that is, CO 2 reduction reaction rate). However, gold is not suitable for large-scale applications owing to its low abundance and high cost. Searching for abundant catalysts with high selectivity is crucial for commercializing CO 2 reduction processes by reducing costs associated with catalyst fabrication and product separation. The selective conversion of CO 2 to CO is a promising route for clean energy. The CO product can be used as feedstock in the Fischer–Tropsch process, a well-known and well-characterized process that has been used in industry to produce chemicals and synthetic fuels from syngas (CO+H 2 ) for many decades [21] . By coupling the catalytic reduction of CO 2 to CO with the Fischer–Tropsch process to produce synthetic fuels and industrial chemicals, the estimated maximum reduction of atmospheric CO 2 emissions is 40% (ref. 22 ). Silver is a promising material as a CO 2 reduction electrocatalyst, because it can reduce CO 2 to CO with a good selectivity (~81%) and it also costs much less than other precious metal catalysts [7] , [23] . In addition, it is expected to be more stable under harsh catalytic environments than homogenous catalysts because of to its all-inorganic nature [13] , [18] . To use its attractive properties, recent research attention has been devoted to developing nanostructured silver-based electrocatalysts with enhanced performance [24] . For example, Rosen et al . [9] reported using Ag nanoparticles as an electrocatalyst in ionic liquid electrolyte (EMIM-BF 4 ) and Salehi-Khojin et al . [25] studied the influence of particle size. An electrocatalytic reduction of CO 2 to CO was observed at an overpotential of 170 mV. However, ionic liquid electrolytes are expensive and sensitive to moisture. Development of CO 2 reduction systems based on aqueous electrolyte with much higher activity is desired for large-scale processes. Here we demonstrate that a nanoporous silver (np-Ag) catalyst is able to reduce CO 2 electrochemically to CO in an efficient and selective manner. Not only does the porous structure create an extremely large surface area for catalytic reaction ( ca. 150 times greater than polycrystalline silver), but also the curved internal surface generates a large number of highly active step sites for CO 2 conversion (at least 20 times more active than polycrystalline silver; Fig. 1a ), resulting in an exceptional activity that is over three orders of magnitude higher than that of the polycrystalline counterpart at a moderate overpotential of <500 mV. More importantly, this CO 2 electroreduction activity has been achieved with a CO Faradaic efficiency of 92%. 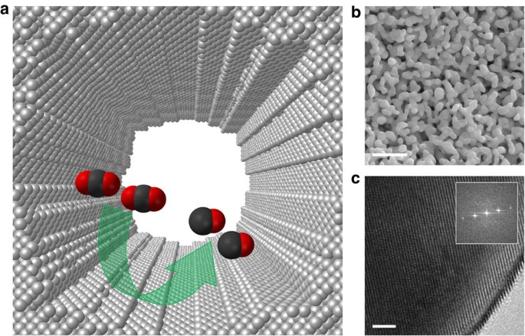Figure 1: Structure and morphology of np-Ag. (a) A schematic diagram of a nanopore of the silver electrocatalyst with highly curved internal surface. (b) Scanning electron micrograph of np-Ag dealloyed in 5 wt% HCl for 15 min and further in 1 wt% HCl for 30 min (scale bar, 500 nm). (c) Corresponding high-resolution transmission electron micrograph with visible lattice fringes. Inset: the Fourier transform shows that the np-Ag is composed of an extended crystalline network (scale bar, 2 nm). Figure 1: Structure and morphology of np-Ag. ( a ) A schematic diagram of a nanopore of the silver electrocatalyst with highly curved internal surface. ( b ) Scanning electron micrograph of np-Ag dealloyed in 5 wt% HCl for 15 min and further in 1 wt% HCl for 30 min (scale bar, 500 nm). ( c ) Corresponding high-resolution transmission electron micrograph with visible lattice fringes. Inset: the Fourier transform shows that the np-Ag is composed of an extended crystalline network (scale bar, 2 nm). Full size image Synthesis and characterization of np-Ag The monolithic np-Ag catalyst was obtained by two-step dealloying of an Ag–Al precursor using an aqueous HCl solution. By selectively etching Al through dealloying, the remaining Ag atoms were reorganized to form a three-dimensional interconnected nanoporous structure. The dealloying process has been reported in a few alloyed systems [26] , [27] and the resulting materials have shown unique catalytic performance such as in fuel cells [28] , [29] , [30] and alcohol oxidation [31] . However, there is still no report on their catalytic properties for CO 2 reduction. A typical scanning electron microscopy (SEM) image of the as-synthesized np-Ag catalyst is shown in Fig. 1b . The ligament size of np-Ag is ~50–200 nm, while the size of the pores extends to a few hundred nanometres. The high-resolution transmission electron micrograph exhibits uniform lattice fringes, and the Fourier transform of the image shows a clear crystallographic symmetry ( Fig. 1c ). Both techniques suggest that the resulting np-Ag is highly crystalline (single-crystal-like), which is further confirmed by powder X-ray diffraction (XRD) data ( Supplementary Fig. 1 ). Additional SEM studies confirm that the resulting nonporous structure is coherent throughout the material (cross-section SEM, Supplementary Fig. 2 ), and no Al residue was detected in either X-ray photoelectron spectroscopy (XPS) ( Supplementary Fig. 3 ) or energy-dispersive spectroscopic analysis. CO 2 reduction performance of the np-Ag catalyst The CO 2 electroreduction activity of np-Ag and polycrystalline Ag was measured using constant-potential electrolysis experiments in a CO 2 -saturated high purity aqueous KHCO 3 electrolyte (0.5 M). In the case of polycrystalline Ag, the electrolyte was treated using a pre-electrolysis process, although no significant difference in activity between treated and untreated electrolytes was observed ( Supplementary Fig. 4 ). Testing was performed in an airtight electrochemical cell with three electrodes and two compartments separated by an anion exchange membrane with electrolyte in each chamber. Gas-phase products from the headspace of the electrochemical cell were measured using gas chromatography (GC) every 30 min. In addition, liquid-phase products were measured using 1 H NMR. CO and hydrogen (H 2 ) were the primary products detected using the GC; however, trace amounts of formate were detected using NMR at potentials more negative than −0.60 V (versus RHE). The electrocatalytic CO 2 reduction results collected at −0.60 V (versus RHE) are presented in Fig. 2a . The geometric current density is calculated based on electrode area. The operating voltage corresponds to an overpotential of 490 mV since the CO 2 /CO equilibrium potential is at −0.11 V versus RHE. At this moderate overpotential, the np-Ag electrode exhibited a long-term stable current of ~18 mA cm −2 during the 2-h electrolytic CO 2 reduction. A high initial current was observed ( Fig. 2a ), which stems from the reduction of a thin surface oxide layer, with an estimated thickness of about 0.5 nm, formed during the material handling in atmospheric air. Faradaic efficiency for CO was maintained at ~92% throughout the electrocatalytic process, further confirming that the np-Ag catalyst was stable under electrocatalytic conditions once the surface oxide layer was removed electrochemically. In a sharp contrast, polycrystalline Ag exhibits a very low current density of 470 μA cm −2 with a poor CO Faradaic efficiency of ~1.1% at the same potential. 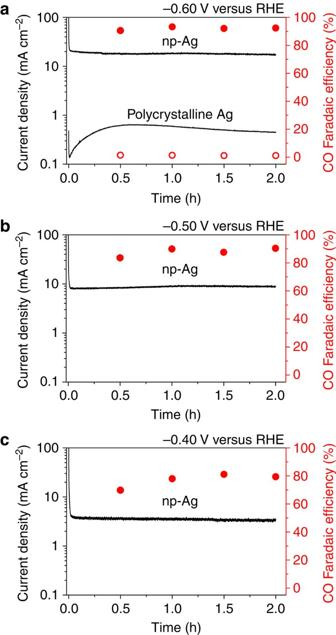Figure 2: Electrocatalytic performance of np-Ag. CO2reduction activity of np-Ag and polycrystalline silver at (a) −0.60 V, and np-Ag at (b) −0.50 V and (c) −0.40 V versus RHE. Total current density versus time on (left axis) and CO Faradaic efficiency versus time (right axis). Figure 2: Electrocatalytic performance of np-Ag. CO 2 reduction activity of np-Ag and polycrystalline silver at ( a ) −0.60 V, and np-Ag at ( b ) −0.50 V and ( c ) −0.40 V versus RHE. Total current density versus time on (left axis) and CO Faradaic efficiency versus time (right axis). Full size image The performances of np-Ag at more positive potentials (−0.50 V and −0.40 V versus RHE, corresponding to overpotentials of 390 mV and 290 mV, respectively) are shown in Fig. 2b,c . With lower overpotentials, smaller currents were observed as expected, while CO Faradaic efficiencies also decreased as potential decreased. At −0.50 V versus RHE, a stable current of ~9.0 mA cm −2 was observed with a CO efficiency of ~90%, whereas at −0.40 V versus RHE a current of ~3.3 mA cm −2 was reached with a CO efficiency of ~79%. The decrease in CO Faradaic corresponds to an increase in the relative rate of hydrogen evolution. This is most likely from the fact that the overpotential is relatively low to drive CO 2 reduction quickly enough to compete with the hydrogen evolution reaction, which only requires a small overpotential to occur. To investigate the maximum CO current density that can be achieved, experiments at higher overpotentials were conducted. The maximum current density of np-Ag for CO production is reached at potentials more negative than −0.8 V versus RHE. A further increase in overpotential does not significantly affect the CO partial current density but instead promotes other product formation (primarily hydrogen but also trace amounts of formate). This can be further seen by the decrease of CO Faradaic efficiency, as potentials are scanned more negative than −0.8 V ( Supplementary Fig. 5 ). Similar behaviour has also been observed in other reports and is most probably due to mass transport limitations of CO 2 at high current densities and not the intrinsic activity of np-Ag [16] , [32] . The structural integrity and surface conditions of post-reacted np-Ag were examined using powder XRD, SEM and XPS techniques. No obvious crystal structure or nanoporous morphology change was observed in either powder XRD ( Supplementary Fig. 1 ) or SEM analysis ( Supplementary Fig. 6 ). The XPS result also revealed that the surface of np-Ag remained stable under these electrocatalytic conditions ( Supplementary Fig. 3 ). To further investigate the long-term stability of the catalytic activity of np-Ag, an 8-h electrolysis was performed under the working condition of −0.50 V (versus RHE). No significant decrease in current density was observed and the CO Faradaic efficiency was maintained above 87% throughout the process ( Supplementary Fig. 7 ). The np-Ag catalyst remained remarkably stable during the extended reaction period, as confirmed by the post-reaction XPS ( Supplementary Fig. 3 ) and SEM ( Supplementary Fig. 7 ) studies. Electrochemical surface area measurement was performed to elucidate the origin of the high activity of np-Ag. The electrochemically active surface area of the np-Ag catalyst was measured by forming an oxide monolayer on the surface electrochemically ( Supplementary Fig. 8 ) [33] . The np-Ag shows an electrochemical surface area (normalized to electrode area) 150 times larger than that of polycrystalline Ag. As the current densities obtained at −0.60 V (versus RHE) for np-Ag is 3,000 times higher than polycrystalline Ag, there is another 20 times difference that cannot be simply explained by the surface area effect alone. This suggests that the intrinsic activity of catalytic sites on the nanoporous surface is much higher than those on a flat surface. Since the activity of np-Ag is mass transport limited at −0.60 V (versus RHE), later shown by the Tafel analysis ( Fig. 3 ), the intrinsic activity for np-Ag is at least 20 times higher than the polycrystalline counterpart. 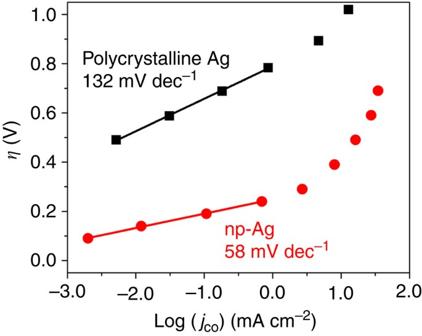Figure 3: Tafel analysis. Overpotential versus CO production partial current density on polycrystalline silver and np-Ag. Figure 3: Tafel analysis. Overpotential versus CO production partial current density on polycrystalline silver and np-Ag. Full size image In addition to polycrystalline Ag, we also compared np-Ag with other Ag nanostructures (for example, nanoparticles and nanowires) as potential CO 2 electrocatalysts ( Supplementary Fig. 9 ). All the experiments were performed under identical conditions (for example, 0.5 M KHCO 3 , pH 7.2 and moderate overpotentials). The results are summarized in Supplementary Table 1 and the typical electrolysis behaviour is shown in Supplementary Fig. 10 . Additional data from recent reports on silver-based CO 2 electrocatalysts have also been included for comparison. The data shown in Supplementary Table 1 and Supplementary Fig. 11 suggest that the np-Ag catalysts in the current work exhibit significant advantages over other silver catalysts under aqueous environments in both overall and per surface site activity. The high performance is attributed to the exposure of the highly active curved internal surface, the greatly enhanced electrochemical surface area and the monolithic self-supported structure with convenient electronic transportation. To explore the kinetics of CO 2 reduction on the np-Ag catalyst surface, Tafel analysis was performed to further determine the intrinsic activity of np-Ag for CO 2 electrocatalytic reduction to CO ( Fig. 3 ). The original data are presented ( Supplementary Fig. 12 and Supplementary Table 2 ). Np-Ag was measured to have a Tafel slope of 58 mV dec −1 compared with 132 mV dec −1 for its polycrystalline counterpart. The sharp decrease of Tafel slope further proves the intrinsically better performance of np-Ag surface. A previous study using single-crystal Ag models by Hori [23] suggested that the stepped Ag (110) surface was more preferred for CO 2 reduction activity than other flat surfaces. It should be noted that such enhancements in np-Ag are achieved at a much lower overpotential than that in single crystal (110) face ( ca. −0.9 V versus RHE). The further improvement in activity may be due to the fact that the np-Ag catalyst contains a higher density of step sites with possibly higher-index facets supported by the highly curved surface [34] , [35] . At higher overpotentials ( η >0.25), a sharp increase of the slope indicates the effect of another rate-limiting step. In this case, the other factor is most probably mass transport issues relating to the diffusion of products and reactants out of/into the nanopores. In addition, mechanistic insight into the two-electron reduction of CO 2 to CO on an Ag surface can be provided from the Tafel analysis [7] . In the first step, one electron is transferred to a CO 2 molecule and forms a CO 2 − intermediate species absorbed on the metal surface. In subsequent steps, the CO 2 − anion takes two protons and another electron, and forms a CO and a H 2 O molecule. Previous studies suggest that the first step proceeds at a much more negative potential than the following steps and is therefore rate determining for the whole process. This is supported by the Tafel slope of 132 mV dec −1 for polycrystalline Ag, close to the calculated value of about 120 mV dec −1 (ref. 36 ). However, for np-Ag, the Tafel slope of 58 mV dec −1 indicates a fast initial electron transfer step before a later non-electron transfer rate-determining step [15] , [36] , [37] , which proves that the np-Ag surfaces are able to stabilize the CO 2 − intermediate much better than a flat surface. Therefore, the dramatic decrease in Tafel slope for np-Ag indicates that, in addition to 150 times larger electrochemical surface area, np-Ag is also intrinsically better than polycrystalline Ag for CO 2 reduction at moderate overpotentials. Further experiments were performed to give greater insight into the mechanism of CO 2 reduction on np-Ag. The dependence of CO 2 reduction activity on CO 2 partial pressure was investigated from 0.1 to 1 atm, which shows an approximate first-order dependence on the concentration of CO 2 in the electrolyte ( Supplementary Fig. 13A ). After the formation of the CO 2 − intermediate, a rate-determining chemical step occurs, followed by a final and relatively fast electron transfer step. A similar study on HCO 3 − concentration shows a zero-order dependence on CO 2 activity, indicating that the donation of a proton from HCO 3 − is not a rate-determining step for CO 2 reduction on Ag surfaces ( Supplementary Fig. 13 ). Another possibility is that the proton is donated from the H 2 O in the electrolyte. However, although the concentration of H 2 O is about 100 times larger than HCO 3 − in the electrolyte, HCO 3 − is actually a more than 10 5 times better hydrogen donor. Therefore, a more likely scenario is that the rate-determining step is not the protonation of CO 2 − intermediate but the surface migration of HCO 3 − to the surface sites inside the pores of np-Ag. With high intrinsic activity, extremely large surface area and superior stability, np-Ag represents the best silver-based electrocatalyst reported so far for CO 2 electroreduction to CO in aqueous electrolyte. The current work has focused on the demonstration of concept and feasibility. The long-term performance of the nanoporous catalyst in a continuous process will be explored using a flow reactor configuration. In addition, mechanical strength of np-Ag may require further investigation before it could be considered in practical applications. Materials Ag–Al precursors were prepared by arc melting pure Ag (Alfa Aesar, 99.9%) and Al (Alfa Aesar, 99.99%) with desired atomic ratio (20:80) under an argon atmosphere. After the verification of composition by energy-dispersive X-ray spectroscopy, the resulting alloy ingot was cut into thin plates with dimensions of 15 × 5 × 0.20 mm 3 using a precision wafering machine. The obtained thin plates were sandwiched between two glass slides and annealed at 546 °C for 12 h to suppress the Ag 2 Al intermetallic compound phase [38] . A rapid cooling process was followed by quenching the thin plates from 546 °C to about 3 °C using a water/ice mixture bath. After the removal of surface rust using sandpaper (240 Grit), pure α-Al(Ag) phase was achieved ( Supplementary Fig. 1 ). The monolithic nanoporous Ag was fabricated by developing a two-step dealloy process. In the first step, the Ag–Al thin plates were immersed into 5 wt% HCl solution as free corrosion for 15 min. Second, the partially leached materials were transferred into 1 wt% HCl solution and dealloyed for about another 30 min until no gas bubbles were produced from the materials. The resulting np-Ag were carefully rinsed with deionized (DI) water for multiple times, dried in vacuum and kept in an Ar-filled glove box under room temperature. Electrodes for electrochemical testing were fabricated by attaching one end of the np-Ag with nickel wires as current collector using silver paint (SPI Supplies). The apparent electrode size used for electrolysis was about 0.25 cm 2 . The polycrystalline Ag electrodes were prepared from Ag foil (Alfa Aesar, 99.998%). The received Ag foil was mechanically polished, etched in sulphuric acid and rinsed with DI water. The apparent electrode size used for electrolysis was about 1 cm 2 . Ag nanoparticle electrodes were prepared by making a suspension with a proportion of 10 mg of Ag nanopowder (<100 nm, Sigma-Aldrich, 99.5% trace metals basis), 600 μl of DI water, 600 μl of isopropyl alcohol and 10 μl of D521 5 wt% nafion solution (DuPont). A following high-power sonication (SONICS Vibra-cell VC 750) was employed to achieve a fine dispersion. The resulting suspension was uniformly coated onto gas diffusion layers of Sigracet 25 BC using a spin coater. Ag nanowire electrodes were prepared in a similar manner. Desired amounts of Ag nanowire (115 nm, Sigma-Aldrich, 0.5 wt% in isopropyl alcohol) were suspended into a mixture to achieve the above proportion of DI water, isopropyl alcohol and nafion. After a rigorous high-power sonication, the suspension was deposited on Sigracet 25 BC gas diffusion layers using a spin coater. After drying in vacuum, the mass loading of Ag materials was determined by comparing the electrode mass before and after the loading process. The apparent electrode size used for electrolysis was about 1 cm 2 . The thickness of the thin oxide layer of np-Ag that formed during the material handling in the atmospheric air was estimated using the following equation: where Q is the amount of charge passed in the first minute of electrolysis at −0.6 V versus RHE, M is molecular weight of Ag 2 O (231.735 g mol −1 ), n is the number of the electron needed to reduce one Ag 2 O molecule, A is the electrode electrochemical surface area, ρ is the density of Ag 2 O (7.14 g cm −3 ) and F is the Faraday constant (9.6485 × 10 4 C mol −1 ). Structural characterization Powder X-ray diffraction (PXRD) patterns were collected using a Rigaku Ultima IV X-ray diffractometer with Cu Kα radiation. Refinement of the PXRD patterns was conducted using the Rietveld approach implemented in Rigaku’s software package PDXL. SEM studies were performed with a JEOL JSM-6330F. High-resolution transmission electron microscopy studies were performed with a JEOL JEM-2010F using an accelerating voltage of 200 kV. X-ray photoelectron spectra were obtained using a Phi 5600 XPS system. Electrochemical characterizations and product analysis A Princeton Applied Research VersaSTAT 3 potentiostat was used for all CO 2 reduction experiments. A piece of platinum wire was used as the counter electrode. The electrolyte was 0.5 M KHCO 3 (Sigma-Aldrich, ≥99.99%) saturated with CO 2 (Matheson, 99.999%) with pH of 7.2. All potentials were measured against an Ag/AgCl reference electrode (3.0 M KCl, BASi) and converted to the RHE reference scale using E (versus RHE)= E (versus Ag/AgCl)+0.210 V+0.0591 × pH. Electrolysis was performed under room temperature in a gas-tight two-compartment electrochemical cell using a piece of anion exchange membrane (fumasep, FAA-3-PK-130) as the separator. Each compartment contained 80.0 ml electrolyte and ~35 ml headspace. Before electrolysis, the electrolyte was purged again with CO 2 gas for at least 30 min and the headspace for at least 20 min. During the electrolysis, the electrolyte in both compartments was stirred at rate of 1,200 r.p.m. using a magnetic stirrer. Gas-phase product was sampled every 30 min using a gas-tight syringe (Hamilton). A gas chromatograph (SHIMADZU, GC-2014) equipped with PLOT MolSieve 5A and Q-bond PLOT columns was used for quantifications. Helium (99.999%) was used as the carrier gas. Liquid product was analysed on a Bruker AVIII 600 MHz NMR spectrometer. A 500-μl electrolyte was sampled at the conclusion of the electrolysis and mixed with 100 μl D 2 O, and 1.67 p.p.m. ( m / m ) dimethyl sulphoxide (Alfa Aesar, ≥99.9%) was added as an internal standard. The one-dimensional 1 H spectrum was measured with water suppression using a presaturation method. For Tafel analysis, CO partial current densities of np-Ag catalyst were averaged over 2 h electrolysis. For polycrystalline Ag, deactivation occurred after 0.5 h and CO activity sharply decreased at potentials more negative than −0.8 V versus RHE; therefore, only initial partial current densities at 0.5 h were used. For testing the CO 2 reduction activity of polycrystalline Ag, a pre-electrolytic process was introduced to further purify the electrolyte because a flat metal surface could be more sensitive to trace amounts of impurities [7] . After a 2-h pre-electrolysis using a sacrificial np-Ag electrode at the same potential as the subsequent test, a freshly prepared electrode was used to measure the CO 2 reduction activity in the conditions described above. The electrochemical surface area measurement was conducted using a beaker-type three-electrode cell equipped with an Ag/AgCl reference electrode (3.0 M KCl, BASi) and a Pt counter electrode. The electrolyte was 0.1 M KOH (Sigma-Aldrich) aqueous solution (N 2 saturated) with pH of 12.6. After electrochemical reduction at −0.4 V (versus RHE) for 10 min, the Ag electrodes were oxidized at 1.15 V (versus RHE), which was believed to only form a monolayer of Ag 2 O or AgOH, corresponding to a charge of about 400 μC cm −2 . By comparing the amount of electrons passed during the oxidation process, the relative surface areas between different Ag electrodes can be obtained ( Supplementary Fig. 8 ) [33] , [39] . The CO 2 partial pressure dependence study was carried out under CO 2 partial pressures ranging from 0.1 to 1.0 atm. A mixture of CO 2 and N 2 gases with the desired ratio was used to purge the cathodic compartment for at least 20 min before electrolysis. A freshly prepared np-Ag electrode was used for electrolysis at each data point and the CO partial current densities were measured at −0.35 V versus RHE. The [HCO 3 − ] dependence study was conducted at concentrations varying from 0.1 to 1.0 M. NaClO 4 (Sigma-Aldrich, 99.99%) was added to the low-concentration electrolytes to keep a same electrolyte ionic strength. A freshly prepared np-Ag electrode was used for electrolysis at each data point and the CO partial current densities were measured at −1.01 V versus Ag/AgCl (corresponding to −0.38 V versus RHE at pH 7.2). How to cite this article: Lu, Q. et al. A selective and efficient electrocatalyst for carbon dioxide reduction. Nat. Commun. 5:3242 doi: 10.1038/ncomms4242 (2014).